Orbital control of western North America atmospheric circulation and climate over two glacial cycles The now arid Great Basin of western North America hosted expansive late Quaternary pluvial lakes, yet the climate forcings that sustained large ice age hydrologic variations remain controversial. Here we present a 175,000 year oxygen isotope record from precisely-dated speleothems that documents a previously unrecognized and highly sensitive link between Great Basin climate and orbital forcing. Our data match the phasing and amplitudes of 65°N summer insolation, including the classic saw-tooth pattern of global ice volume and on-time terminations. Together with the observation of cold conditions during the marine isotope substage 5d glacial inception, our data document a strong precessional-scale Milankovitch forcing of southwestern paleoclimate. Because the expansion of pluvial lakes was associated with cold glacial conditions, the reappearance of large lakes in the Great Basin is unlikely until ca. 55,000 years into the future as climate remains in a mild non-glacial state over the next half eccentricity cycle. Paleoclimate proxy data from marine sediments, polar ice cores and cave deposits have revealed an orbital pacing that linked global ice volume, atmospheric greenhouse gas concentrations, polar temperatures, and monsoon strength over several ice age cycles [1] , [2] , [3] . In contrast, the paleoclimatic evolution of mid-latitude continental regions is less well understood because few records have sufficient dating control, duration, and temporal resolution to compare with orbital-scale climate variations. In particular, the Devils Hole, Nevada, calcite δ 18 O record [4] has led to interpretations that western North America ( Fig. 1 ) responded asynchronously with Northern Hemisphere summer insolation, calling into question the applicability of Milankovitch forcing to explain paleoclimate there. 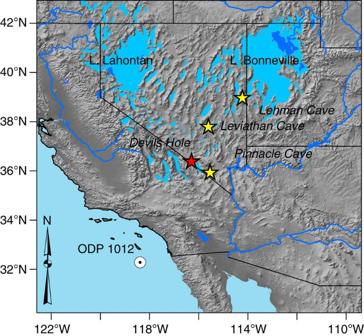Figure 1: Study areas in the Great Basin. Map shows southwestern North America with location of pluvial lakes and sites mentioned in text. Stalagmite LC-1 was recovered from Leviathan Cave, stalagmite PC-1 was collected from Pinnacle Cave, and stalagmites LMC-14, LMC-21, and LC-2 of ref.25were collected from Lehman Cave. Figure 1: Study areas in the Great Basin. Map shows southwestern North America with location of pluvial lakes and sites mentioned in text. Stalagmite LC-1 was recovered from Leviathan Cave, stalagmite PC-1 was collected from Pinnacle Cave, and stalagmites LMC-14, LMC-21, and LC-2 of ref. 25 were collected from Lehman Cave. Full size image Despite the poor understanding of orbital-scale forcing on pluvial lake cycles, abundant evidence of large late Quaternary lakes attests to the sensitivity of Great Basin hydrology to ice age climate changes [5] . Prominently, lakes Lahontan and Bonneville reached large extents near the end of the last ice age 25-15 ka (ka=thousands of years before present) [6] , [7] . Geomorphic evidence of dramatic lake level changes attests to large hydrological variations occurring over millennial time scales, yet constraining climate variations from lake deposits alone is complicated by fragmentary preservation, long periods of slow or non-deposition during non-pluvial conditions [8] , [9] , uncertain reservoir effects on carbonate 14 C dating [10] , and the inherent limits on radiocarbon dating to less than ca. 45 ka (ref. 11 ). The Milankovitch theory of ice ages [1] posits that ice-sheet growth occurred over tens of thousands of years by the accumulation of high-latitude snow as a result of sufficiently low Northern Hemisphere summer insolation at 65°N (hereafter ‘summer insolation’), and is supported by an orbital pacing of global ice volume [2] and a large body of other paleoclimatic data [12] . Rapid glacial retreat is attributed to rising summer insolation, ice-sheet instability and feedbacks associated with rising sea level, vegetation change, increased Southern Ocean upwelling and concomitant rising atmospheric CO 2 concentrations [13] . Expanded ice sheets had widespread global impacts via changes in atmospheric circulation and temperature [12] , and have been linked to pluvial lake-filling episodes during glacial marine isotope stages (MIS) [7] , [8] . We use these stages here, defined by the ice volume proxy of marine benthic δ 18 O values, as a convenient shorthand for contemporaneous variations in other orbital and terrestrial paleoclimate parameters. A major advance in the study of Great Basin paleoclimate was achieved with the Devils Hole oxygen isotopic (δ 18 O) record [14] , [15] , [16] of subaqueous calcite lining the walls of an open fault zone within the regional groundwater aquifer, and allowed the first continuous paleoclimate record that could be radiometrically dated beyond the reach of radiocarbon (50 ka). Devils Hole thereby provided a test of the nature and timing of previous glacials/interglacials between 500 to 4 ka (refs 4 , 14 ). However, the Devils Hole record presented a paradox because it appeared to show deglacial warming that preceded orbital forcing [14] and global ice volume terminations [2] by thousands of years. The origin of this asynchrony has been debated for several decades [17] , [18] , [19] , [20] , [21] , [22] , [23] . Although the Devils Hole δ 18 O time series is still cited as a challenge to Milankovitch forcing [24] , one attempt to reconcile Devils Hole and orbital theory involved reconstructions of sea surface temperatures along the western margin of North America associated with fluctuations in the strength of the California Current [21] . Here, SST increases also preceded global ice volume terminations, likely driven by interactions between near-coastal waters and North American ice-sheet extent, thus apparently removing Devils Hole as a fundamental challenge to Milankovitch theory [20] , [21] , but it also now leaves the question of climate forcing open. Because the existing temperature records suggested that western North America paleoclimate was asynchronous with orbital variations, major questions remain as to the nature and timing of glacial/interglacial warmings, the duration of interglacial periods, and the relationship between orbital forcing and pluvial lake expansion in the Great Basin. Moreover, the early warming events observed in the Devils Hole and California margin records are anomalous relative to other terrestrial paleoclimate data [8] , [23] that suggest Great Basin paleoclimate varied coherently with global ice ages. In particular, speleothem records from Pinnacle [23] and Lehman Caves [25] , Nevada, indicated glacial and deglacial timings that were consistent with Milankovitch forcing, thus calling again into question the nature of Devils Hole calcite as a record of Great Basin climate [22] , [26] . However, these stalagmite time series were short (~5,000 years), and no other long-term Great Basin vadose zone speleothem records were previously available to corroborate their timing or that of Devils Hole. To address the timing of paleoclimate change and its implications for Milankovitch forcing, we present a new Great Basin stalagmite δ 18 O record (hereafter ‘δ 18 O-GB’) from vadose zone (above the water table) caves spanning the past 175,000 years. Vadose zone speleothems have a more straightforward relationship to infiltration pathways and flow times than phreatic zone calcite, making their link to surface climate more direct. From these deposits we show evidence for a strong orbital forcing of Great Basin paleoclimate over the last 175,000 years. Age dating and oxygen isotopic time series The new speleothem reconstruction ( Fig. 2 and Supplementary Fig. 1 ) is anchored by 65 precise U-Th dates ( Supplementary Table 1 and Supplementary Fig. 2 ) and 1,936 δ 18 O measurements, and is supplemented by a published Lehman Cave speleothem record [25] . The reconstruction is based on records from three Great Basin caves with differing drip-water δ 18 O values, so the records were normalized to a common δ 18 O scale (see Methods). Because modern precipitation δ 18 O values ( Supplementary Fig. 3 ) are strongly correlated with temperature both temporally and spatially ( Supplementary Fig. 4 ) and are inversely correlated to the latitude of moisture source [27] , we interpret δ 18 O-GB as a proxy for temperature and moisture source of winter precipitation reaching the Great Basin. The δ 18 O values of atmospheric moisture reflect rainout history at and upwind of the precipitation site over a wide geographic area [28] , and these winter precipitation δ 18 O variations are subsequently transmitted to caves [23] , [29] as drip waters where they are recorded in speleothem calcite. 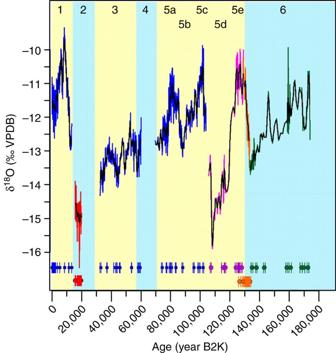Figure 2: Great Basin paleoclimate record. High-resolution δ18O time series (top) and precise U-series ages±two sigma (bottom) from Nevada Cave stalagmites LC-1 (blue), PC-1 (red), LMC-14 (magenta), LC-2 of ref.25(orange) and LMC-21 (Green). Numbers along top indicate Marine Isotope Stages. The data are normalized for site latitude and corrected for changes in ocean δ18O. The δ18O-GB time series shows a saw-tooth structure over the last two glacial cycles that is interpreted as a paleotemperature and moisture source δ18O proxy for southwestern North America that varies on orbital time scales. Black line is a 750-year running average to emphasize trends. Figure 2: Great Basin paleoclimate record. High-resolution δ 18 O time series (top) and precise U-series ages±two sigma (bottom) from Nevada Cave stalagmites LC-1 (blue), PC-1 (red), LMC-14 (magenta), LC-2 of ref. 25 (orange) and LMC-21 (Green). Numbers along top indicate Marine Isotope Stages. The data are normalized for site latitude and corrected for changes in ocean δ 18 O. The δ 18 O-GB time series shows a saw-tooth structure over the last two glacial cycles that is interpreted as a paleotemperature and moisture source δ 18 O proxy for southwestern North America that varies on orbital time scales. Black line is a 750-year running average to emphasize trends. Full size image Great Basin paleoclimate linked to orbital insolation Our results provide strong support for a Milankovitch forcing of Great Basin paleoclimate over the past 175,000 years. Our data show strong correspondence to June 21–August 21 insolation at 65°N ( Fig. 3 ), and exhibit a one-to-one match of peak δ 18 O and low ice volume that defines the classic saw-tooth pattern of ice age cycles. There is a remarkable coherency in the timing of δ 18 O variability among the samples collected from three caves spread across thousands of square kilometres ( Fig. 1 ). Most prominently, δ 18 O-GB variations show a remarkable fit of relative peak and trough amplitudes to the obliquity- and eccentricity-modulated 23-kyr precession cycle of summer insolation. The interhemispheric correspondence between the δ 18 O-GB and globally distributed climate records is evident in matched high δ 18 O-GB values and increased temperature [30] and methane concentrations in the Antarctic EPICA Dome C ice core [31] and shared variations with benthic foraminifera δ 18 O values [2] , a proxy for global ice volume. These correlations support our interpretation that δ 18 O-GB is a proxy for past temperature and atmospheric circulation. Interestingly, our data do not show the pronounced millennial-scale climate variations evident in other southwestern speleothem records [32] , [33] over MIS 3, so we focus on the orbital-scale variations. This discrepancy may indicate that the northern limit of summer moisture penetration into the Great Basin was south of our study area, or because of varying seasonal sensitivity at our site relative to New Mexico and Arizona. 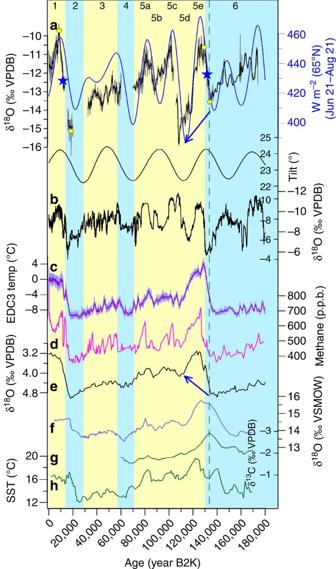Figure 3: Comparison of Great Basin and global paleoclimate records. ais the Great Basin δ18O record plotted with summer insolation integrated over June 21–August 21 for 65°N and obliquity (tilt) variations;bis the δ18O record of the Asian Monsoon (two y-axes reflect different caves);canddare the temperature and CH4records from the EPICA (Antarctica) Dome C ice core, respectively;eis the LR04 benthic foraminifera δ18O stack, a proxy for global ice volume;fis Devils Hole δ18O; G is Devils Hole δ13C on an inverted axis, and H is the California margin SST (core ODP 1012). Numbers at top indicate Marine Isotope Stages. Blue arrows show contrasting MIS 6 and 5d signals for δ18O-GB and insolation (top) and ice volume (benthic δ18O, bottom). The ages of the half-height δ18O-GB rises (blue stars) around ice volume Terminations I and II were based on the minimum and maximum δ18O values (yellow circles); δ18O values above the half-height rise indicate interstadial warmth. The vertical dashed green line indicates timing of Devils Hole δ13C minimum, which coincides with minimum δ18O-GB and supports a cold and wet pluvial climate during the penultimate glacial maximum. Figure 3: Comparison of Great Basin and global paleoclimate records. a is the Great Basin δ 18 O record plotted with summer insolation integrated over June 21–August 21 for 65°N and obliquity (tilt) variations; b is the δ 18 O record of the Asian Monsoon (two y-axes reflect different caves); c and d are the temperature and CH 4 records from the EPICA (Antarctica) Dome C ice core, respectively; e is the LR04 benthic foraminifera δ 18 O stack, a proxy for global ice volume; f is Devils Hole δ 18 O; G is Devils Hole δ 13 C on an inverted axis, and H is the California margin SST (core ODP 1012). Numbers at top indicate Marine Isotope Stages. Blue arrows show contrasting MIS 6 and 5d signals for δ 18 O-GB and insolation (top) and ice volume (benthic δ 18 O, bottom). The ages of the half-height δ 18 O-GB rises (blue stars) around ice volume Terminations I and II were based on the minimum and maximum δ 18 O values (yellow circles); δ 18 O values above the half-height rise indicate interstadial warmth. The vertical dashed green line indicates timing of Devils Hole δ 13 C minimum, which coincides with minimum δ 18 O-GB and supports a cold and wet pluvial climate during the penultimate glacial maximum. Full size image Timing and duration of Great Basin interglacials Our data further show the expected timing of glacial-interglacial transitions associated with rising summer insolation, and that MIS 5 was characterized by a triple peak in δ 18 O during substages 5a, 5c and 5e ( Fig. 3 ). We estimated the timings of Great Basin glacial-interglacial transitions around global ice volume Terminations I and II (TI and TII) from the timing of δ 18 O-GB half-height increases. The TII δ 18 O-GB rise robustly constrains a half-height age of 131.8 ka, which is within age uncertainties of TII (131.6 ka) in the orbitally tuned global ice volume record [2] and confirms the timing estimated previously from the short Lehman Cave record [25] . Because of the exceptional U-series age precision on the stalagmites LC-14 and LC-21 of better than±0.4%, the timing of the δ 18 O-GB half-height rise at TII is tightly constrained. The TI half-height rise in δ 18 O-GB is less well constrained because of non-growth intervals in our record (see Supplementary Discussion ), but was estimated to 11.9 ka by using the 18.6 ka δ 18 O-GB minimum and peak Holocene warming at ca. 8.55 ka. This timing may be too young, and its true age is likely closer to that estimated from continuous growth speleothems from Arizona [33] and New Mexico [32] at 15.0 and 14.8 ka, respectively. Low δ 18 O-GB values (cold conditions) during the last and penultimate glacial maxima coincide with minima in Antarctic temperature and maximal ice volume as would be expected from Milankovitch forcing, but contrast with warm California margin alkenone-based SSTs. Our data show that the duration of MIS 5e warmth in the Great Basin is 10.9 kyr (between 131.8 to 120.9 ka), as defined by δ 18 O-GB exceeding the glacial to interglacial half-height of −12.1‰, ( Fig. 3 ). The ~11 kyr duration is consistent with that inferred from summer insolation, global ice volume and Antarctic ice cores [30] , [31] , but is significantly shorter than the 22-kyr interglacial inferred from Devils Hole [4] , [34] . Further, δ 18 O-GB shows a return to interglacial warmth during MIS 5a and 5c, similar to the triple peak interglacial observed in the Asian monsoon [3] and Antarctic methane records, as would be expected from a summer insolation forcing. The MIS 5 triple peak contrasts with relatively less pronounced MIS 5c and 5a warmings in Antarctic temperature and CO 2 , providing evidence that summer insolation was a dominant control on Great Basin paleoclimate. Holocene North Atlantic imprints Our data also show similarities to Holocene climate variations in the North Atlantic region: low δ 18 O values indicate cool conditions at 12.5 ka during the Younger Dryas (YD), to attainment of peak warming at 8.6 ka, similar to Greenland temperature ( Fig. 4 ). High-speleothem δ 13 C values further support the inference of dry conditions during the YD and early Holocene [35] , [36] ( Fig. 4 and Supplementary Fig. 5 ) because soil carbonate δ 13 C is inversely correlated with rainfall amounts in the Great Basin via a soil productivity forcing [37] . A trend to cooler and moister late Holocene climate is evident in decreasing δ 18 O values and faster stalagmite growth rates, which peak around 3–5 ka, an observation consistent with similar changes in the Southwest [36] but contrasting with apparent climate stability in Greenland [38] and Devils Hole [4] . This transition to wetter climates and more productive soils beginning ca. 5 ka may have facilitated the growth of the ancient 4.9 ka bristlecone pine [39] stand on the flank of Wheeler Peak, Nevada. Further, we observe a strong inverse correspondence between δ 18 O-GB values and the strength of the East Asian Summer Monsoon [40] (Dongge Cave, China) over the past 13 kyr, confirming that the trans-Pacific climate synchrony previously observed for the Southwest and Asia on the millennial-scale [32] extends to the Great Basin on orbital time scales. 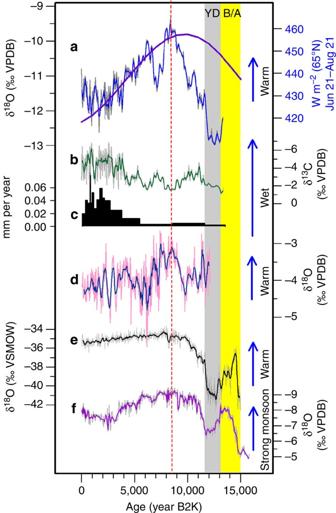Figure 4: Holocene North Atlantic imprints. Detail of the last 15 kyr show imprints of orbital insolation and North Atlantic climate variability on Great Basin paleoclimate.ais Great Basin stalagmite LC-1 δ18O with 150-year running average plotted with 65°N summer insolation;bis LC-1 δ13C values with 150-year running average;cis stalagmite growth rate;dis Pink Panther Cave stalagmite δ18O, New Mexico;eis NGRIP Greenland δ18O record on the GICC05 timescale;fis Donnge Cave (Asian Monsoon) speleothem δ18O; B/A is the Bolling/Allerod warm period; YD is the Younger Dryas cold event. Vertical dashed red line indicates peak Great Basin warmth at 8.5 ka that lags peak summer insolation at 11 ka. Figure 4: Holocene North Atlantic imprints. Detail of the last 15 kyr show imprints of orbital insolation and North Atlantic climate variability on Great Basin paleoclimate. a is Great Basin stalagmite LC-1 δ 18 O with 150-year running average plotted with 65°N summer insolation; b is LC-1 δ 13 C values with 150-year running average; c is stalagmite growth rate; d is Pink Panther Cave stalagmite δ 18 O, New Mexico; e is NGRIP Greenland δ 18 O record on the GICC05 timescale; f is Donnge Cave (Asian Monsoon) speleothem δ 18 O; B/A is the Bolling/Allerod warm period; YD is the Younger Dryas cold event. Vertical dashed red line indicates peak Great Basin warmth at 8.5 ka that lags peak summer insolation at 11 ka. Full size image Pluvial Lake expansion and Great Basin paleoclimate The GB-δ 18 O time series sheds light on the origin of the Great Basin’s pluvial lakes. A remarkable correlation between GB-δ 18 O values and the level of Lake Lahontan [41] ( Fig. 5 ) shows that lake high stands were associated with lowest speleothem δ 18 O values between 20 and 14 ka, and lowest lake levels with high δ 18 O values, for example, around 8 ka. Maximum lake levels during cold periods thus were supplied by high-latitude moisture derived from a northerly source region. This observation is consistent with fresh conditions and inferred high-latitude moisture filling lakes in southern California [42] , but not with the hypothesis of a tropical moisture source [41] . Low lake levels coincided with dry and warm conditions during the early Holocene which then shifted towards slightly cooler and wetter conditions in the late Holocene associated with the Fallon Lake cycles in the Lahontan Basin [7] . Given the strong inverse correlation between stalagmite δ 18 O and pluvial lake level over the past 25,000 years, our new 175,000 year δ 18 O-GB record suggests that similar pluvial lake expansions may have occurred during other cool periods as documented for MIS 2 at Pyramid Lake [43] , for MIS 3 cool events in Lake Bonneville [10] , during the penultimate glacial maximum (MIS 6), and perhaps during MIS 5d when δ 18 O values reach minimum values, consistent with correlations of deep lake cycles with glacial maxima [7] , [8] . 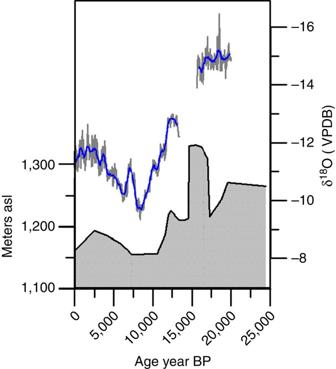Figure 5: Correlation of Great Basin pluvial lake and climate. Correlation between δ18O-GB and Lake Lahontan level shows speleothem δ18O values (blue line) are inversely correlated to pluvial lake size (grey fill—note inverted oxygen isotope axis). We conclude that lake expansions were associated with colder and/or a higher latitude moisture source. Figure 5: Correlation of Great Basin pluvial lake and climate. Correlation between δ 18 O-GB and Lake Lahontan level shows speleothem δ 18 O values (blue line) are inversely correlated to pluvial lake size (grey fill—note inverted oxygen isotope axis). We conclude that lake expansions were associated with colder and/or a higher latitude moisture source. Full size image Our data document a previously unrecognized and robust link between Great Basin climate and summer insolation. The saw-tooth character of the δ 18 O-GB record over the past 175 ka suggests that global ice volume and insolation are first-order controls on western North America paleoclimate. On a finer temporal scale, the amplitudes and phasing between δ 18 O-GB and summer insolation provide two important clues for Great Basin climate attribution. First, sequentially lower insolation minima (cooling) centred on 138 ka (MIS 6) and 114 ka (MIS 5d) are mimicked by correlative speleothem δ 18 O ( Fig. 3 ), but contrast with relative ice volume maxima that show a warming trend from MIS 6 to MIS 5d. The MIS 6 δ 18 O-GB low happens during rising obliquity and warming Northern Hemisphere summers, which may have diminished cooling relative to MIS 5d, when obliquity and δ 18 O-GB were low. Further correspondence is evident in a matched triple peak of warming (high δ 18 O-GB) in marine isotope substages 5a, 5c and 5e that follows summer insolation and is similar to the triple peaks of methane [31] in Antarctic ice and strong monsoon intervals in Asia [3] , but contrasts with increasing ice volume, and decreasing Antarctic temperature and CO 2 levels. The greater similarity of δ 18 O-GB to precessional-scale variations in summer insolation than to global ice volume, particularly during MIS 5, suggests a fast-response forcing on precipitation δ 18 O variations. A second clue is the observation that δ 18 O-GB minima lag insolation minima by ca. 3 kyr (significantly exceeding age uncertainties) at the MIS 6/5 and 2/1 transitions, reaching minima at 134 and 18.6 ka, respectively, compared with insolation minima at 137 and 22 ka. The lags suggest that summer insolation did not directly force atmospheric temperature (for example, via heating of the atmosphere by more intense summer insolation), but must have acted indirectly by another mechanism. We argue that the fast-response forcing of δ 18 O-GB resulted from atmospheric circulation anomalies driven by variations in Northern Hemisphere sea ice, continental snow cover and incipient ice-sheet growth that responded to summer insolation [44] . Periods of low summer insolation would have allowed persistence of summer snow (for example, during MIS 5d), which in turn likely affected the delivery of high-latitude precipitation during cold periods, and vice versa. Changes in winter moisture source may have also resulted in temperature anomalies from the ice-albedo feedback to produce our observed δ 18 O-GB record. The lags in δ 18 O-GB minima after insolation suggest that several millennia of snow and ice accumulation past the insolation minimum were required before exerting a maximal influence on North Pacific storm tracks. In turn, these circulation anomalies drove the expansion and contraction of Great Basin pluvial lakes during cold and warm conditions, respectively, thus allowing for correlation and future projection of high-lake level stands to low insolation. Additional tests of the climate/lake level correlation, such as during MIS two and three [10] await further high-resolution lake level dating and continuous speleothem data over this time interval. Our data provide additional evidence for the importance of MIS 5d for glacial inception [44] over North America during an interval of low obliquity ( Fig. 2 ). The MIS 5d orbital configuration has been hypothesized to be a key forcing of the initiation of Northern Hemisphere glaciations, and would have driven the expansion of Arctic sea ice and perennial snow cover. Initial ice build up during MIS 5d was volumetrically small with a concomitant minor change in benthic δ 18 O, but an areally-extensive snow cover could have strongly impacted circulation patterns via atmospheric and land-surface albedo feedbacks [44] . Climate simulations set to 115 ka obliquity values found that when perihelion occurs during the northern winter, reduced summer insolation allows snow to persist through the summer [44] , resulting in a stronger Aleutian Low [45] and strengthened storm tracks [46] over the eastern North Pacific, supported by δ 18 O-GB minima during MIS 5d. Consistent with observations of the development of atmospheric circulation anomalies following ice-sheet growth [47] , we suggest that the low δ 18 O values around MIS 5d may be related to the development of a stationary wave that resulted in transmission of low-δ 18 O moisture to the study area. Our data provide evidence that the last glacial inception may have been partly triggered by cold atmospheric conditions during MIS 5d in western North America, and provide a challenge to test whether climate models are capable of reproducing our observations of rapid precessional-scale climate variability at times of low ice volume. Despite several decades of controversy on the forcings of Great Basin paleoclimate, our new data show that atmospheric circulation over the northeastern Pacific Ocean and Great Basin was indeed paced by Milankovitch forcing. Our new data support previous interpretations that the Devils Hole δ 18 O record may have been influenced by changing latitudes of infiltration of ground water into the regional carbonate aquifer reaching Devils Hole [23] . Variable proportions of higher latitude and altitude ( ca. 38°N) waters with low δ 18 O values and lower latitude ( ca. 36°N) higher δ 18 O waters could have influenced the shape of the Devils Hole δ 18 O curve. If the proportion of low-latitude ground waters reaching Devils Hole varied significantly ~10 kyr before global ice volume terminations, it would have produced a δ 18 O increase that mimicked an early deglacial warming. Although this mechanism is speculative, it could be tested by additional work on fluid inclusions of both the Devils Hole phreatic calcite and our vadose zone speleothems, and more high-resolution dating of the Devils Hole phreatic calcite. Our data demonstrate that Great Basin stalagmite δ 18 O variations closely match the shape and amplitudes of 65°N summer insolation, documenting a strong Milankovitch forcing on southwestern paleoclimate. We have shown that this orbital control is linked to the expansion of pluvial lakes during full glacial periods. Because the ongoing interglacial appears most analogous to the very long ‘super interglacial’ [48] of MIS 11 (424–374 ka), and because modern warming (increasing δ 18 O-GB) appears to have already begun despite decreasing summer insolation, we hypothesize that future climate variations will also follow summer insolation. Rising insolation and an added anthropogenic climate control is likely to keep Great Basin climate mostly mild [49] and dry [50] over the next half eccentricity cycle until insolation reaches a new minimum ~55,000 years in the future ( Fig. 6 ). 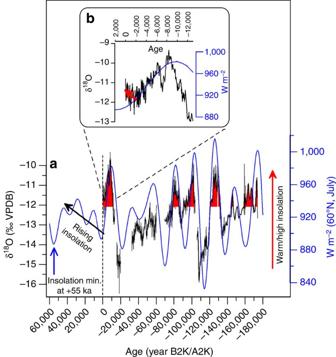Figure 6: Projection of western North America paleoclimate. ashows the strong link between July insolation at 60°N latitude and Great Basin δ18O values over the past 175,000 years, and projection of rising insolation (black arrow) suggests continued non-glacial conditions over the next half eccentricity cycle until insolation reaches a minimum in about 55,000 years A2k (after year 2,000 CE; blue arrow).bis inset showing that Great Basin warming began about 1,600 years ago (linear fit shown as red arrow) when insolation was still declining. Figure 6: Projection of western North America paleoclimate. a shows the strong link between July insolation at 60°N latitude and Great Basin δ 18 O values over the past 175,000 years, and projection of rising insolation (black arrow) suggests continued non-glacial conditions over the next half eccentricity cycle until insolation reaches a minimum in about 55,000 years A2k (after year 2,000 CE; blue arrow). b is inset showing that Great Basin warming began about 1,600 years ago (linear fit shown as red arrow) when insolation was still declining. Full size image Study area The three caves in our study area are located in the central Great Basin: Leviathan Cave is located in the Worthington Mountains (37.89°N, 115.58°W, 2,400 m) of Nevada, in the northern part of the Death Valley regional ground water flow system that also feeds Devils Hole. Stalagmite LC-1 was collected from this cave and covers the YD to modern and portions of MIS 3 and MIS 5. The sampling site has constant temperature (8.32±0.06 °C) and 100% relative humidity, based on 23 months of continuous data logging (27-May-2011 to 28-April-2013). Stalagmite LC-1 was collected beneath an active drip and is 551 mm tall. Stalagmite PC-1 was collected from Pinnacle Cave (35.97°N, 115.50°W, 1,792 m), on the flank of Mount Potosi in the Spring Mountains of southern Nevada. The entrance to Pinnacle Cave is restricted and requires a long vertical drop, ensuring the cave has a stable cave climate and high-relative humidity. Pinnacle Cave is located in the Spring Mountain recharge zone for Devils Hole; details on Pinnacle Cave and stalagmite PC-1 were previously reported [23] . Lehman Cave is located in Great Basin National Park (39.0°N, −114.2°W, 2,080 m). Stalagmites LMC-14 and LMC-21 were collected down and broken from deep within Lehman Cave. Additionally, we used the recently-published data for stalagmite LC-2 from Lehman Cave [25] . The LC-2 stalagmite represents a key time interval of Termination II and connects a temporal gap between our LMC-14 and -21 stalagmites, and we confirm that it records climate variations in the Great Basin over the penultimate termination [25] . The hydrology of the alpine cave sites is straightforward, as they each receive water from infiltration of precipitation through overlying bedrock and are not connected to regional aquifers. Each of the caves is overlain by only a few tens of metres of overlying carbonate bedrock, and because of their ridge-top locations, they receive water infiltration only from directly above the drip sites. Because of these characteristics, the selected cave drip hydrology can be considered a more robust proxy for δ 18 O of precipitation than groundwater-fed vein calcite, which integrates isotope signals over large areal and latitudinal extents. Isotopic analyses U-series ages were determined at the Radiogenic Isotope Laboratory, University of New Mexico, by dissolving subsample powders (50–200 mg) in nitric acid and spiking them with a mixed 229 Th- 233 U- 236 U spike. The U and Th isotopic measurements were made on a Thermo Neptune Plus multi-collector inductively coupled plasma mass spectrometer. Analytical uncertainties are 2σ of the mean; age uncertainties include analytical errors and uncertainties in the initial 230 Th/ 232 Th ratios, which is set equal to 4.4 p.p.m. by assuming a bulk earth 232 Th/ 238 U value of 3.8. U-series ages ( Supplementary Table 1 ; Supplementary Fig. 2 ) are in correct stratigraphic order (except for one closely-spaced age pair at 60 and 64 mm in LMC-14, which have identical ages within uncertainty), and have high precisions, in most cases better than ±1%. The stalagmite age models in years before 2,000 CE (year B2k) were determined from linear interpolation between dates; for the minor (within uncertainty) age inversion in LMC-14, the 60-mm subsample was omitted from the linear age model. δ 18 O subsamples were drilled or milled from the growth axis at intervals ranging from 0.1 to 1.0 mm, resulting in an average sub-decadal to centennial-scale time resolution. δ 18 O values were analyzed at the Las Vegas Isotope Science Lab, University of Nevada Las Vegas, by phosphoric acid reaction at 70 °C in a Kiel IV automated carbonate preparation device coupled to a ThermoElectron Delta V Plus mass spectrometer, and corrected with internal and external standards. δ 18 O and δ 13 C precisions are better than 0.08‰. δ 18 O and δ 13 C are defined as δ=( R sample − R standard )÷ R standard × 1,000, where R is the ratio of 18 O/ 16 O and 13 C/ 12 C in per mil (‰) variations of the sample relative to the Vienna Pee Dee Belemnite (VPDB) standard ( δ =0‰ for both oxygen and carbon). Stable isotopic data will be deposited at the NOAA Palaeoclimatology data repository at http://www.ncdc.noaa.gov/paleo/paleo.html . Composite time series A composite δ 18 O time series was constructed by interpolating the measured δ 18 O time series ( Supplementary Fig. S1 ) at a 50 year resolution and splicing into a single time series by choosing the record of highest temporal resolution, best dating or most continuous coverage (‘Measured’ time series in Supplementary Fig. S1 ). Then, the composite time series was corrected for changes in the δ 18 O value of the ocean [51] (‘Sea-water corrected’). Lastly, because the three cave sites span 340 km of latitude and have site-water (precipitation) δ 18 O values that decrease by ca. 3‰ with increasing latitude, the δ 18 O data were normalized by the different site-water δ 18 O values to plot on the same δ 18 O scale as LC-1. This normalization was realized via multiple regression, using winter precipitation-amount weighted δ 18 O values from the central Great Basin [52] , supplemented with stable isotopic data of creeks and springs near Lehman Cave in Great Basin National Park [53] , [54] . The multiple regression model contained two significant ( P -value <0.05) variables: latitude (in decimal degrees) and altitude (in metres) to yield the equation δ 18 O=(latitude × −0.593718666)+(altitude × −0.001075451)+9.773431178 ( r 2 =0.65; RMSE=0.93; P -value =0.00022). The model has a median δ 18 O residual of ±0.62‰, indicating high-predictive power. The model resulted in δ 18 O values, relative to Leviathan Cave, of -0.36‰ at Lehman Cave, and +1.73‰ at Pinnacle Cave, and the δ 18 O time series for Lehman and Pinnacle Caves were thus adjusted by these offset amounts (‘Sea and site-water corrected’ time series in Supplementary Fig. 1 ). This offset correction allows for the direct comparison of the δ 18 O values between the sites. The resulting time series spans 174,100 years, with gaps between 13,350 and 15,650, 20,050 and 32,300, 60,150 and 69,650 and 103,800 and 105,700 years before 2,000 CE (year B2k). year B2k, respectively. The age models ( Supplementary Fig. S2 ) are expressed in yr B2k. Assessment of isotopic equilibrium Stalagmite LC-1, the only stalagmite that was actively growing when collected, is in apparent isotopic equilibrium with cave drip water. Using the equation of (ref. 55 ), a temperature of 8.3 °C, and average δ 18 O value of calcite deposited over the last 200 years of −11.56‰ VPDB, the drip-water δ 18 O value with which the calcite is in isotopic equilibrium is −14.24‰ Vienna standard mean ocean water (VSMOW), which is identical to measured drip-water δ 18 O value of -14.23‰ VSMOW. The Leviathan, Pinnacle and Lehman Cave drip water and spring isotope values plot directly on the southern Nevada winter meteoric water line ( Supplementary Fig. S3 ), indicating they are unaffected by evaporation. The low-drip-water δ 18 O values of between -12 and -14‰ VSMOW indicate a winter precipitation source, consistent with mountain recharge in the Great Basin [23] , [29] . Stable-isotope values in modern precipitation Winter precipitation, falling mostly as snow, is the dominant source of groundwater recharge in the Great Basin [29] . To determine the correlation between winter precipitation δ 18 O and climate variables, we extracted a sub-set of 18 stations with winter δ 18 O values from the Friedman et al. analysis [52] , supplemented by data for Great Basin National Park. We determined the Pearson correlation coefficients and significance levels in Microsoft Excel between precipitation-weighted winter δ 18 O values at each site to average winter temperature and precipitation over the months of December–April extracted from the WorldClim database [56] for each site location. The average winter temperatures were calculated as the median values of the average-minimum and -maximum temperatures. These data ( Supplementary Fig. 4 ) show a statistically-significant and strong correlation between winter δ 18 O and median temperature (δ 18 O=0.31 × Temp (DJFMA) −15.78, r =0.82, P <0.000005, n =19), but no significant correlation to precipitation amount ( r =−0.35, P =0.14). This spatial correlation shows that temperature is a strong and dominant control on the δ 18 O values of mean winter precipitation. This spatial δ 18 O temperature effect has a temporal corollary whereby winter precipitation δ 18 O values are inversely related to the origination latitude of source moisture, with low δ 18 O values associated with a northerly (cold) moisture source in the Gulf of Alaska, and highest values with a subtropical (warm) Pacific source [27] . Further, a detailed analysis of regional event-based δ 18 O of precipitation demonstrated that the lowest at-a-site δ 18 O values had moisture sources around 50°N, whereas the highest δ 18 O values had a moisture source at around 20°N in the tropical Pacific Ocean [57] , demonstrating that the temporal variations in δ 18 O at individual locations varies strongly as a function of moisture source. Additional discussion is included in [22] , [26] . Although the modern Δδ 18 O/ ΔT gradient is well constrained both spatially (Δδ 18 O/ΔT=0.31‰ / °C) and temporally (Δδ 18 O/ΔT=0.96‰ / °C), we do not quantitatively interpret the δ 18 O time series in terms of temperature, because (1) it is unclear which of the two Δδ 18 O/ΔT gradients is more relevant, and (2) the Δδ 18 O/ΔT gradients may have changed over time under different climatic boundary conditions, as has been demonstrated at other sites [58] . However, the strong correlation between δ 18 O and temperature reflects the fundamental processes of Rayleigh distillation and moisture source origination, such that colder moisture sources (for example, Gulf of Alaska) and colder atmospheric temperatures result in lower δ 18 O values, and our data is highly correlated to summer insolation in a sense expected by the temperature effect. As such, we favour a semi-quantitative interpretation of speleothem δ 18 O values as a paleotemperature and moisture source proxy. How to cite this article: Lachniet, M. S. et al. Orbital control of Western North America atmospheric circulation and climate over two glacial cycles. Nat. Commun. 5:3805 doi: 10.1038/ncomms4805 (2014).